DNA origami based assembly of gold nanoparticle dimers for surface-enhanced Raman scattering Plasmonic sensors are extremely promising candidates for label-free single-molecule analysis but require exquisite control over the physical arrangement of metallic nanostructures. Here we employ self-assembly based on the DNA origami technique for accurate positioning of individual gold nanoparticles. Our innovative design leads to strong plasmonic coupling between two 40 nm gold nanoparticles reproducibly held with gaps of 3.3±1 nm. This is confirmed through far field scattering measurements on individual dimers which reveal a significant red shift in the plasmonic resonance peaks, consistent with the high dielectric environment due to the surrounding DNA. We use surface-enhanced Raman scattering (SERS) to demonstrate local field enhancements of several orders of magnitude through detection of a small number of dye molecules as well as short single-stranded DNA oligonucleotides. This demonstrates that DNA origami is a powerful tool for the high-yield creation of SERS-active nanoparticle assemblies with reliable sub-5 nm gap sizes. Structural DNA nanotechnology [1] and in particular DNA origami [2] has emerged as a versatile ‘bottom-up’ approach for the assembly of both two- and three-dimensional nanostructures with tailored geometries [3] , [4] . Such structures have been typically assembled by folding a long ‘scaffold’ strand of viral single-stranded DNA (ssDNA) using multiple short ssDNA ‘staple’ strands; however, they can also be assembled without the use of a scaffold [5] , [6] , [7] . The strength of this technique has been demonstrated in a number of applications including control and study of molecular transport in cells [8] , [9] , [10] , drug delivery systems [11] , as platforms for single-molecule chemical reactions [12] , [13] , rulers for super-resolution microscopy [14] , [15] as well as nanopore biosensors [16] , [17] , [18] . Furthermore, the double helical structure of DNA offers the possibility of unique binding sites with a regular spacing of ~7 nm (21 bp) along the helix and ~3 nm perpendicular to the helical axis [19] which makes DNA origami perfectly suited as a platform for the assembly of multi-component nanostructures [20] , [21] . A particularly exciting sensing application utilizing plasmons has been the creation of metallic nanostructures using double-stranded DNA (dsDNA) linkers [22] , [23] as well as DNA origami [24] . The oscillations of conduction electrons create localized surface plasmons in metal nanoparticles (NPs) which enhance local fields in a small volume around the NP [25] , [26] . Much DNA assembly work has therefore focused on creating precise geometries to harness novel optical behaviour emerging from the coupling of NP surface plasmons in chiral assemblies [27] , [28] , [29] . However, while these properties have been demonstrated using bulk measurements such as circular dichroism or ultraviolet–visible spectrometry, there have been only a few studies carefully characterizing the plasmonic properties of single nanostructures [30] which reveals the crucially important uniformity in the assembly process. For future applications of DNA-based assemblies, characterization of the effect of DNA origami on the plasmonic properties of NP assemblies is thus essential. DNA origami-assembled NP dimers are also promising for single-molecule spectroscopic techniques such as surface-enhanced fluorescence [31] , as demonstrated by Acuna et al. [32] In that work, a DNA origami pillar with docking sites was used for assembly of NP dimers separated by 23 nm. The structures yielded an average enhancement factor of 28 in the fluorescence emission of a dye molecule embedded within the DNA pillar. These plasmonic nanoantennas have potential for single-molecule Förster resonance energy transfer assays or protein-binding assays; however, the analytes need to be labelled and embedded within the origami pillar and the structures produce a large range of enhancement factors. A label-free alternative to enhanced fluorescence is surface-enhanced Raman scattering (SERS) [33] , [34] . Because Raman scattering cross-sections are typically 10 orders of magnitude smaller than fluorescence cross-sections [35] , a much larger enhancement factor is required. This makes these dimers based on DNA origami pillars unsuitable for SERS measurements. Here we report the successful assembly of 40 nm Au NP dimers with sub-5 nm gaps on a 40 × 45 nm 2 DNA origami platform ( Fig. 1a ). The innovative design of the origami platform ensures a strong plasmonic coupling between the NPs without occupying the gap between them. Using these structures, we are able to address the specific issues described earlier. Far field scattering measurements of individual structures unveils a significant red shift in the plasmonic resonances due to the underlying DNA origami platform, as well as their consistent architecture. The strong optical coupling allows us to demonstrate SERS measurements of both an external analyte as well as ssDNA oligos attached to the NPs using these structures. 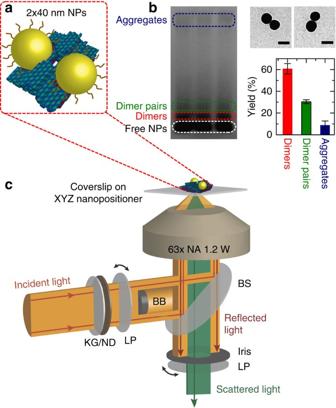Figure 1: Overview of the experimental set-up. (a) A schematic (not to scale) of the NP dimers assembled on the DNA origami platform. The NPs are coated with a ssDNA brush to prevent aggregation as well as facilitate attachment to the origami platform. (b) Correctly formed dimer structures are separated from free NPs and aggregates by gel electrophoresis on a 0.7% agarose gel and imaged using a TEM (scale bar, 50 nm). The yield of these structures is around 61±5% (mean±s.d.) as measured by the intensity of the dimer and aggregate bands. (c) A schematic of the custom built setup for measuring the scattering spectra of single dimer nanostructures. KG: heat absorbing filter; ND: neutral density filter; LP: linear polarizer; BB: beam block; and BS: beam splitter. Figure 1: Overview of the experimental set-up. ( a ) A schematic (not to scale) of the NP dimers assembled on the DNA origami platform. The NPs are coated with a ssDNA brush to prevent aggregation as well as facilitate attachment to the origami platform. ( b ) Correctly formed dimer structures are separated from free NPs and aggregates by gel electrophoresis on a 0.7% agarose gel and imaged using a TEM (scale bar, 50 nm). The yield of these structures is around 61±5% (mean±s.d.) as measured by the intensity of the dimer and aggregate bands. ( c ) A schematic of the custom built setup for measuring the scattering spectra of single dimer nanostructures. KG: heat absorbing filter; ND: neutral density filter; LP: linear polarizer; BB: beam block; and BS: beam splitter. Full size image Assembly of NP dimers with a sub-5 nm gap An overview of the experimental scheme is depicted in Fig. 1 . A multi-layer 40 × 45 nm 2 DNA origami platform is assembled as described in Methods section. By varying the number of layers along the origami structure, two grooves are created to facilitate the correct positioning of two 40 nm Au NPs. These grooves are separated and isolated from each other by a ridge of double helices. At its highest the ridge is six helices (~15 nm) high. Crucially, in the gap directly between the NPs, the ridge is only two helices (~5 nm) thick, which leaves the gap free for utilization of single-molecule spectroscopic techniques. Gold NPs are attached to correctly folded origami structures using a protocol given in Kuzyk et al. [27] Agarose gel electrophoresis is used to isolate the dimers from aggregates and incorrectly assembled structures as well as the large excess of free NPs. Based on an intensity analysis of the dimer and aggregate bands in Fig. 1b , the yield is 61±5%. While a small number of structures with only one NP attached are present within the dimer band, these are easily identifiable from the dimers due to their dramatically different spectral response. From transmission electron microscope (TEM) images of correctly assembled structures ( Fig. 1b ), we measure an average NP separation of 3.3±1.0 nm which is one of the shortest controllable gaps yet achieved with DNA origami assembly. Characterization of plasmonic properties We examined carefully the contributions of individual components of the assembled nanostructures to the plasmonic resonance of the NPs. A supercontinuum laser was employed in a reflective dark-field geometry to collect far-field scattering spectra of individual structures ( Fig. 1c ) [36] , [37] . We obtained spectra from both individual ssDNA-coated NPs as well as single ssDNA-coated NPs attached to a flat DNA origami sheet and immobilized on a poly-( L )-lysine-coated glass slide. Heat absorbing and neutral density filters were used to ensure radiant flux densities are below the damage threshold of the DNA origami structures. In all cases, the presence of the DNA changes the dielectric properties of the environment around the NPs, allowing an effective refractive index for both layers to be calculated [38] . Three representative spectra for single ssDNA-coated NPs are shown in Fig. 2a , their similar intensities are further verification of consistent single NP measurements. The peak intensity of these NPs ( Fig. 2c ) already displays an average red shift of 6±1 nm (mean ± s.e.) from bare NPs on glass (scattering peak at 530±1 nm, data shown in Supplementary Fig. 1 ). From TEM images, the thickness of the ssDNA coating was found to be 2.5±0.5 nm. This value was used in numerical simulations ( Supplementary Fig. 2 ) to estimate the effective refractive index n ssDNA of the ssDNA layer. A value of n ssDNA =1.7±0.1 was found to best fit the measured spectra ( Fig. 2b , Supplementary Figs 3 and 4 , Supplementary Notes 1 and 2 ). 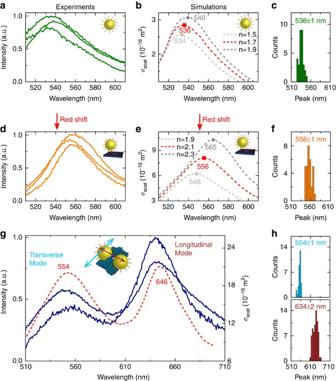Figure 2: Effective refractive index for DNA origami nanostructures. Simulations for the scattering cross-section are presented in (b,e), the other panels are experimental data. Errors quoted are s.e. of the mean. A single peak is obtained for ssDNA-coated NPs (a) with an average red shift of 6±1 nm from the bare NP peak (c). This corresponds to an effective refractive index ofnssDNA=1.7 (b). A single peak (d) with a further red shift of 20±1 nm is obtained for single nssDNA-coated NPs attached to flat origami sheets (f). UsingnssDNA=1.7 from (b), the best fit is obtained fornorigami=2.1 (e). The two peaks for the NP dimer structures (g) correspond to the transverse and longitudinal modes. The overlaid scattering cross-section obtained from simulations (red dashed line, no free parameters) has peaks at 554 and 646 nm, in good agreement with the experimental data (g,h). Figure 2: Effective refractive index for DNA origami nanostructures. Simulations for the scattering cross-section are presented in ( b , e ), the other panels are experimental data. Errors quoted are s.e. of the mean. A single peak is obtained for ssDNA-coated NPs ( a ) with an average red shift of 6±1 nm from the bare NP peak ( c ). This corresponds to an effective refractive index of n ssDNA =1.7 ( b ). A single peak ( d ) with a further red shift of 20±1 nm is obtained for single nssDNA-coated NPs attached to flat origami sheets ( f ). Using n ssDNA =1.7 from ( b ), the best fit is obtained for n origami =2.1 ( e ). The two peaks for the NP dimer structures ( g ) correspond to the transverse and longitudinal modes. The overlaid scattering cross-section obtained from simulations (red dashed line, no free parameters) has peaks at 554 and 646 nm, in good agreement with the experimental data ( g , h ). Full size image The controlled attachment of single ssDNA-coated NPs to flat DNA origami sheets allowed for the characterization of any red shift caused by the DNA origami sheet and subsequent extraction of the effective refractive index of DNA origami. Binding of single NPs was achieved by designing an origami sheet with sufficient DNA docking sites for only a single NP. A lower NP: origami ratio was used and the monomers were carefully isolated using gel electrophoresis. Once again, the scattering intensities are similar for each nanostructure ( Fig. 2d ). The scattering peaks also display a more pronounced red shift ( Fig. 2f ) of 20±1 nm and 26±1 nm as compared with the peaks for ssDNA-coated ( Fig. 2c ) and bare NPs ( Supplementary Fig. 1 ), respectively. This increased red shift is clearly attributable to the underlying origami structure ( Supplementary Note 3 ). To simplify the simulations, the underlying origami sheet was modelled as an infinite lateral sheet of 5 nm thickness, with the ssDNA coating described by n ssDNA =1.7. The best fit to the experimental data was obtained for n origami =2.1 ( Fig. 2e , Supplementary Fig. 4 , Supplementary Note 4 ). Given the density of the DNA in the sheet compared with the ssDNA on the particles, this increased effective n origami =2.1±0.05 is not surprising. Finally, individual dimer structures were characterized. Correctly assembled dimers were easily identifiable due to their characteristic polarization-dependent response and enhanced scattering ( Fig. 2g and Supplementary Fig. 5 ). Typically, the longitudinal mode (excited by light polarized along the dimer axis) is expected to be strongly red-shifted due to the plasmonic coupling between the NPs, whereas the transverse mode (light polarized perpendicular to the dimer axis) should remain nearly unchanged from the single NP resonance [35] . Indeed as clearly evident, the transverse mode peak for NP dimer structures ( Fig. 2g,h ) coincides almost exactly with the scattering peak for single ssDNA-coated NPs on origami sheets ( Fig. 2d,f ). The two parameter values n ssDNA =1.7 and n origami =2.1 were used to simulate the scattering cross-section of the dimer structures. The dimers were modelled as a pair of NPs covered with a 2.5 nm thick ssDNA layer separated by 3.3 nm on an infinite origami sheet of 5 nm thickness. The simulations are shown by the red-dashed line in Fig. 2g and are in very good agreement with the experimental data ( Fig. 2h ). Our values of n origami =2.1 and n ssDNA =1.7 are very similar to those reported for 54 bp ( n =2.1) and 24 bp ( n =1.75) long dsDNA coating around 20 nm gold NPs, also measured using plasmon resonances [38] . We also repeated all scattering measurements with the structures surrounded by buffer instead of air ( Supplementary Fig. 6 ). The resonance peak for ssDNA-coated NPs is red-shifted by 5±1 nm, as expected given the higher refractive index of water compared with air. However, for single ssDNA-coated NPs on flat DNA origami sheets, no shift in the resonance peak is observed, whereas for the dimer structures, the longitudinal mode is blue-shifted by 10±2 nm. This blue shift, despite the increased refractive index of water as surrounding medium could be caused by an increase in spacing between the NPs as the ssDNA coating gets hydrated ( Supplementary Fig. 7 ). These measurements are further proof of the strong plasmonic coupling in our dimer structures, and that the architecture can be controlled by flexing of the DNA origami under appropriate stimulation. SERS measurements of external analytes After the careful characterization of our dimer structures, we investigated their potential for SERS measurements of external analytes. Individual dimer structures are immobilized on a gold-coated silicon wafer as described in Methods. The gold coating reduces background Raman emissions from the silicon wafer. The immobilized dimer structures are incubated briefly in a 100 μM solution of Rhodamine 6G to form a monolayer on the dimer structures ( Fig. 3a ) before the solution is removed [39] . Rhodamine 6G is a model Raman analyte with many characteristic peaks [40] . SERS measurements were carried out with a Renishaw inVia Raman microscope using a 100 × objective with NA=0.85. Laser-induced damage to the dimers was prevented by illuminating with low intensities (see Supplementary Fig. 8 ). The spectra were taken on individual dimers which can be identified on the gold surface. A collection of spectra, each obtained from a different dimer structure are shown in Fig. 3b . Typical Rhodamine 6G modes common to all spectra are highlighted by red-dashed lines. We employed a laser excitation line at 632.8 nm, which is in close proximity to the longitudinal dimer mode ( Fig. 2c ). Hence, the observed enhancement is highly sensitive to the polarization of the laser with respect to the dimer axis ( Supplementary Fig. 9 ). Assuming a monolayer coverage [41] of Rhodamine 6G (density of 10 −13 molecules cm −2 ) on the NP and the corresponding sensing volume of 10 −25 m −3 , there should be around five molecules contributing to the SERS signal (see Supplementary Methods ). Depending on the orientation of the dimer in the laser field, we calculate surface enhancement factors between five and seven orders of magnitude. This is in good agreement with our simulations (see Supplementary Fig. 10 ) and in line with other SERS systems [35] . Similar results are obtained for other external analytes as shown in Supplementary Fig. 11 . Away from the NP (marked as ‘off dimer’ in Fig. 3b ), the Raman spectrum of the Rhodamine is completely absent for the concentrations used. 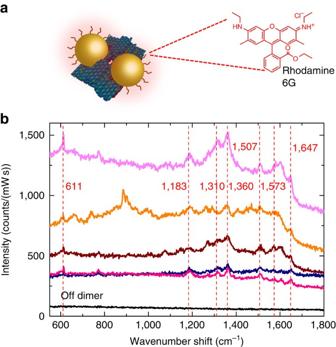Figure 3: SERS measurements of an external analyte. (a) SERS measurements of a thin layer of Rhodamine 6G adsorbed onto individual dimer structures plated on a gold-coated silicon wafer. (b) Each spectrum corresponds to a different dimer structure and typical Rhodamine 6G peaks are clearly visible (indicated by a dashed line). By contrast, a spectrum taken from a region away from the dimers (‘off dimers’) is of low intensity and does not display any peaks. Figure 3: SERS measurements of an external analyte. ( a ) SERS measurements of a thin layer of Rhodamine 6G adsorbed onto individual dimer structures plated on a gold-coated silicon wafer. ( b ) Each spectrum corresponds to a different dimer structure and typical Rhodamine 6G peaks are clearly visible (indicated by a dashed line). By contrast, a spectrum taken from a region away from the dimers (‘off dimers’) is of low intensity and does not display any peaks. Full size image Sequence-specific DNA detection using SERS A powerful application of our dimer structures would be to combine the binding site possibilities of the origami platform with label-free SERS detection. To demonstrate this, we performed SERS measurements on individual dimer structures without any externally added analyte in a similar manner as described above. The gap between the NPs is free except for the ssDNA coating. Measurements were first performed with NPs coated with 19 bases of Thymine (‘sequence 1’). Typical data for a range of dimers are shown in Fig. 4b . The peak at 1,000 cm −1 is thought to arise from the in-plane rocking mode in Thymine [42] , and the peak at 1,084 cm −1 corresponds to the phosphate backbone of DNA [42] , [43] . An additional peak at 1,576 cm −1 may arise from the 15 bp poly-Adenine sequence (complementary to the ssDNA coating on the NPs) on the origami platform used for NP attachment [43] . To investigate if we could detect changes in the oligonucleotide sequence, dimer structures were assembled from a mixture of 80% ‘sequence 2’ containing Cytosine and Adenine in addition to Thymine and 20% ‘sequence 1’, as shown in the schematic in Fig. 4 . This combination ensured enough of sequence 1 was present in order to attach the NPs to the DNA origami platform. As can be seen in Fig. 4c , peaks for Adenine (736, 1,260 and 1,485 cm −1 ) [43] and Cytosine (1,260 and 1,485 cm −1 ) [44] are now observed in addition to the peaks already marked in Fig. 4b . 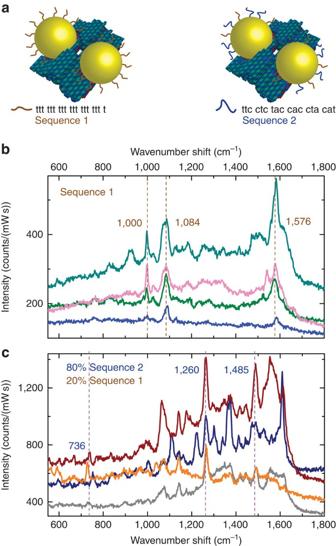Figure 4: SERS spectra are sensitive to the sequences of the ssDNA coating. (a,b) The ssDNA coating of 19 bases of Thymine (‘sequence 1’) on the NPs produces spectra with peaks predominantly corresponding to the DNA backbone (1,000 cm−1) and Thymine (1,084 cm−1), indicated by the red dashed lines. (b,c) By contrast, the use of an Adenine and Cytosine containing ‘sequence 2’ in an 80:20 ratio with ‘sequence 1’ shows significantly more peaks corresponding to Adenine (736, 1,260 and 1,485 cm−1) and Cytosine (1,260 and 1,485 cm−1), indicated by the blue dashed lines. Figure 4: SERS spectra are sensitive to the sequences of the ssDNA coating. ( a , b ) The ssDNA coating of 19 bases of Thymine (‘sequence 1’) on the NPs produces spectra with peaks predominantly corresponding to the DNA backbone (1,000 cm −1 ) and Thymine (1,084 cm −1 ), indicated by the red dashed lines. ( b , c ) By contrast, the use of an Adenine and Cytosine containing ‘sequence 2’ in an 80:20 ratio with ‘sequence 1’ shows significantly more peaks corresponding to Adenine (736, 1,260 and 1,485 cm −1 ) and Cytosine (1,260 and 1,485 cm −1 ), indicated by the blue dashed lines. Full size image Once again, in comparison with bulk Raman measurements of the same oligos, we obtain an average enhancement of 4–5 orders of magnitude in the scattering cross-section if we assume that a single DNA molecule with around 20 bases is present in the sensing volume. Such a consistently high enhancement factor demonstrates the potential these structures have for label-free single-molecule measurements such as sequence-sensitive DNA detection in combination with high-throughput techniques. The presence of a strong plasmonic gap built over a customisable DNA origami platform makes it an exciting prospect for hybrid plasmonic nanopores and many other DNA-based probes. In summary, DNA origami offers an elegant approach to design metallic nanostructures with complex optical properties. In this paper, we demonstrate an innovative origami design that allows for the reliable assembly of 40 nm Au NP dimer structures with strong plasmonic coupling from reliable sub-5 nm gaps. This is reflected in the high uniformity of scattering spectra of individual dimers which obey the characteristic polarization-dependent response of strongly coupled NPs. We are also able to demonstrate that the underlying DNA origami platform has a significant influence on the plasmonic properties of the dimer. The effective refractive index for dense DNA origami estimated from finite-difference time-domain (FDTD) simulations is in good agreement with similar measurements for dsDNA on gold NPs. We demonstrate the effectiveness of our dimer structures for SERS measurements with enhancement factors of up to seven orders of magnitude. We are able to detect not only external analytes with only a handful of adsorbed molecules in the sub-5 nm, but also changes in the composition of the ssDNA coating on the NPs. This effectively demonstrates the combination of a versatile platform for biosensing (DNA origami) with a label-free detection technique (SERS) and has great potential application for a wide variety of biosensing and single-molecule applications. DNA origami structure design and assembly All DNA origami structures were designed using the open source DNA origami software caDNAnano [45] . All short ssDNA staples were purchased from Integrated DNA Technologies. The precise sequence of staples for as well as the scaffold/staple layout for each design are included Supplementary Tables 1 and 2 and Supplementary Figs 12 and 13 . The flat origami design used for attachment of single NPs in Fig. 2b consists of a double layer with 24 interlinked double-helical DNA domains on each layer on a square packing lattice. Eight staples on one layer included ssDNA overhangs for attachment to complementary ssDNA on the NPs. These were organized into two distinct binding sites comprised of four staples each with different ssDNA overhangs; ttt ttt ttt ttt ttt (complementary to ‘sequence 1’) and atg tag gtg gta gag g (complementary to ‘sequence 2’). Consequently, NPs coated with sequence 1 ssDNA could only attach to the staples on one of the binding sites. The 7,249 bases of viral M13mp18 ssDNA was utilized as the scaffold (New England Biolabs). DNA origami assembly was done by mixing scaffold and staples to a final concentration of 10 nM and 100 nM, respectively, in a 14 mM MgCl 2 solution buffered with 1 × TE (pH=8.0) and subjecting the mixture to thermal-annealing cycles for 18 h. The heating program utilized was as described in Hernández-Ainsa et al. [46] The NP dimer design consists of multiple layers of double-helical DNA domains on a square packing lattice such that a ridge of DNA seven helices (17.5 nm thick) separates two large grooves custom designed to fit 40 nm NPs. In each groove, six staples are modified to include overhangs complementary to sequence 1. The p8634 mutant of the viral M13 genome was utilized as the scaffold and the structure requires 251 staple strands of DNA. DNA origami assembly was carried out in a similar fashion as described above, with a modified thermal annealing programme was follows: 80 °C for 5 min, 79 °C for 4 min, from 79–60 °C in 19 steps (1 °C per step, 4 min each step), 60 °C for 12 min, from 60 to 15 °C in 90 steps (0.5 °C per step, 12 min each step) and finally set at 4 °C. The assembled structures were purified from the excess staple strands by centrifugation with 100 kDa MWCO filters (Amicon Ultra, Millipore) in three cycles at a speed of 13,000 g for 5 min at 4 °C in a 0.5 × TBE buffered solution of 11 mM MgCl 2 . The assembled origami structures were then collected at the end of the third cycle of filtration. ssDNA coating of NPs and synthesis of dimer structures A detailed attachment protocol is given in Kuzyk et al. [27] Briefly, 40 nm gold NPs (BBI Solutions) are resuspended in 2.5 mM Bis (p-sulfonatophenyl)phenylphosphine dihydrate dipotassium (BSPP) solution (Sigma Aldritch) to enable higher NP concentrations. DNA oligos corresponding to ‘sequence 1’ or ‘sequence 2’ are ordered with a 5′ dithiol modification (Biomers). After incubation in 10 mM Tris(2-carboxyethyl)phosphine (TCEP, Sigma Aldritch) for 30 min, they are added in a 4,800-fold excess to the NP solution. Following a protocol given in Zhang et al. [47] , citrate-HCl buffer (pH=3) is added to a final concentration of 10 mM for 10 min, before HEPES buffer (pH=7) is added at a final concentration of 100 mM. This protocol ensures quick attachment of thiolated ssDNA oligos to the gold NPs. Successful attachment is confirmed by a lack of aggregation when resuspended in 100 mM MgCl 2 . ssDNA-coated NPs are separated from excess DNA oligos by eight rounds of centrifugation with 100 kDa MWCO filters (Amicon Ultra, Millipore) at 10,000 g for 10 min at 4 °C and finally incubated overnight with the assembled DNA origami platforms in a 0.5 × TBE buffered solution of 11 mM MgCl 2 so that the NPs are in a 10 × excess per binding site. Successful formation of dimers and separation from larger aggregates is accomplished by gel electrophresis in a 0.7% agarose gel run at 60 V and maintained at 4 °C by a surrounding ice bath. Immobilization of dimers on glass or gold-coated Si wafer Glass coverslips (Academy) are plasma cleaned (air plasma treatment at 100 W plasma power in a Femto-Diener Electronic plasma cleaner) for 10 min to ensure hydrophilicity and activation of the silane groups and one side is covered with a 1 mg ml −l solution of poly-( L )-lysine (Sigma Aldritch) for 2 min. The coverslips are then washed twice with distilled water and then the same side is covered with a dilute solution of assembled dimer structures in 11 mM MgCl 2 solution buffered with 0.5 × TBE for a further 2 min. The coverslip surface is then further washed with distilled water and then air dried with a nitrogen gun to ensure a uniform coverage of dimer structures. Flat gold surfaces are prepared by electron-beam evaporation of a 5 nm chromium adhesion film on a silicon wafer followed by 70 nm of gold (the evaporation rate is kept below 0.5 nm). For the immobilization of dimer structures on these wafers, the plasma cleaning step is omitted. Scattering spectroscopy Scattering spectra were taken on a custom built inverted microscopy setup which employs a Fianium SC400-4 supercontinuum laser (400–1,700 nm) as illumination source. The inner part of the beam is blocked and the remaining light sent through the outer part of a bright-field objective (Leica HPX Plan APO 63x NA 1.2 W). The scattered light is collected through the centre of the objective lens and sent to an OceanOptics QE65000 spectrometer for analysis. Numerical simulations FDTD calculations were carried out with Lumerical FDTD v8.6 and structures modelled as shown in Supplementary Fig. 2 . The ssDNA layer was modelled as a 2.5 nm thin dielectric coating of the Au NP. For simplicity, DNA origami and glass coverslips were implemented as semi-infinite half-space with a constant real dielectric constant. Illumination with s and p polarized plane waves was performed at an angle of incidence of 60° to replicate the axial polarization component used in the experimental dark-field illumination. The resulting spectra were added incoherently to obtain the scattering cross-section for illumination with unpolarized light. How to cite this article: Thacker, V. V. et al. DNA origami based assembly of gold nanoparticle dimers for surface-enhanced Raman scattering. Nat. Commun. 5:3448 doi: 10.1038/ncomms4448 (2014).